Clinical implications of genomic alterations in the tumour and circulation of pancreatic cancer patients Pancreatic adenocarcinoma has the worst mortality of any solid cancer. In this study, to evaluate the clinical implications of genomic alterations in this tumour type, we perform whole-exome analyses of 24 tumours, targeted genomic analyses of 77 tumours, and use non-invasive approaches to examine tumour-specific mutations in the circulation of these patients. These analyses reveal somatic mutations in chromatin-regulating genes MLL , MLL2 , MLL3 and ARID1A in 20% of patients that are associated with improved survival. We observe alterations in genes with potential therapeutic utility in over a third of cases. Liquid biopsy analyses demonstrate that 43% of patients with localized disease have detectable circulating tumour DNA (ctDNA) at diagnosis. Detection of ctDNA after resection predicts clinical relapse and poor outcome, with recurrence by ctDNA detected 6.5 months earlier than with CT imaging. These observations provide genetic predictors of outcome in pancreatic cancer and have implications for new avenues of therapeutic intervention. Worldwide, over 250,000 patients develop pancreatic ductal adenocarcinoma every year and a vast majority die of their disease [1] . Pancreatic ductal adenocarcinoma comprises ∼ 85% of all pancreatic neoplasms, with ∼ 60–70% of cancers localized to the head of the pancreas, 20–25% in the body or tail and the remaining cases involving the entire organ [2] . Currently, surgical resection of the tumour is the only potentially curative treatment. However, only a minority (15–20%) of patients are candidates for pancreatectomy at the time of diagnosis [3] . This can largely be attributed to the fact that pancreatic cancer develops over decades as a result of the accumulation of genetic mutations and other molecular abnormalities and clinical presentation often occurs very late in the history of the disease [4] . The 5-year survival rate for those diagnosed with pancreatic cancer remains <10% (ref. 1 ). Several genetic alterations have been identified in pancreatic cancers, including those in the CDKN2A , SMAD4 and TP53 tumour suppressor genes, and in the KRAS oncogene [5] , [6] . Although the discoveries of these genes and their pathways have provided important insights into the natural history of pancreatic cancer and have spurred efforts to develop improved diagnostic and therapeutic agents, few genetic alterations discovered to date in pancreatic cancer have been used to directly affect clinical care [1] , [7] . To identify genetic alterations that may be related to patient outcome and other clinical characteristics, we performed large-scale genomic analyses of pancreatic adenocarcinomas using two prospectively collected clinical cohorts. These analyses revealed somatic mutations in chromatin-regulating genes as well as in genes with potential clinical utility using existing or experimental therapies. We also used liquid biopsy approaches to evaluate circulating tumour DNA (ctDNA) for non-invasive detection of early-stage pancreatic cancer as well as for identifying recurrent or residual disease. Taken together, these analyses provide predictors of clinical outcome in pancreatic cancer and have implications for personalized therapeutic intervention in these patients. Next-generation sequencing analyses of pancreatic cancer We used next-generation sequencing to examine the entire exomes of matched tumour and normal specimens from 24 patients and targeted sequencing to analyse an additional 77 patient tumours. These approaches allowed us to identify sequence changes, including single base and small insertion or deletion mutations, as well as copy number alterations in >20,000 genes in the whole-exome analyses and in 116 specific genes in the targeted analyses ( Fig. 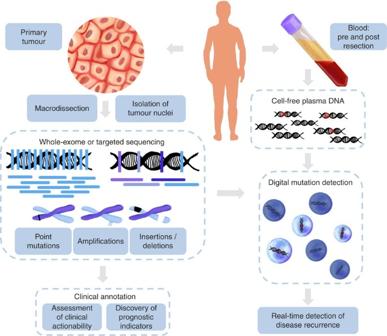Figure 1: Schematic of next-generation sequencing and ctDNA analyses. Next-generation sequencing analyses were performed for tumour specimens obtained from pancreatic ductal adenocarcinoma patients using either whole-exome or targeted analyses focused on 116 genes. Genomic alterations were evaluated for potential clinical utility or as prognostic indicators. Somatic mutations identified through genomic analyses were used to evaluate patient plasma for detection of ctDNA at the time of diagnosis or after surgical intervention. 1 and Supplementary Table 1 ). The pancreatic cancers analysed were stage II tumours in patients who underwent potentially curative resections ( Supplementary Data 1 ). Given the low neoplastic cellularity of pancreatic cancers [5] , we enriched for neoplastic cells either by macrodissecting primary tumours or by flow-sorting tumour nuclei, and performed high-coverage sequencing of these enriched samples. We obtained a per-base sequencing coverage of 234-fold for each tumour analysed by whole-exome sequencing and 754-fold for each tumour analysed by targeted cancer gene sequencing (Methods, Supplementary Data 2 ). Figure 1: Schematic of next-generation sequencing and ctDNA analyses. Next-generation sequencing analyses were performed for tumour specimens obtained from pancreatic ductal adenocarcinoma patients using either whole-exome or targeted analyses focused on 116 genes. Genomic alterations were evaluated for potential clinical utility or as prognostic indicators. Somatic mutations identified through genomic analyses were used to evaluate patient plasma for detection of ctDNA at the time of diagnosis or after surgical intervention. Full size image Using a high-sensitivity mutation detection pipeline [8] , we detected an average of 114 tumour-specific (somatic) non-synonymous sequence alterations in the cancers analysed by whole-exome sequencing, similar to previous studies of this tumour type [5] , [6] , and 4.7 non-synonymous sequence alterations per cancer in the targeted analyses ( Supplementary Data 3 ). 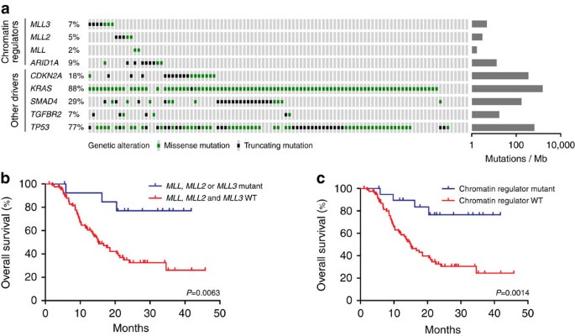Figure 2: Recurrent genetic alterations in pancreatic cancer and their effect on disease outcome. (a) Representation of the mutations identified in chromatin modifying and other recurrently mutated genes. Each patient sample is indicated as a grey box with mutations indicated in green or black. (b) Analyses of overall survival revealed that patients wild type for MLL gene alterations (n=87) had a significantly lower median survival compared with those with mutated MLL genes (n=14; median survival 15.3 months versus not reached respectively,P=0.0063, log-rank test). (c) Similar analyses revealed significantly improved survival in patients with mutations in eitherMLLorARID1Agenes (n=20) compared with those that were wild type for any of these genes (n=81). Among known recurrent sequence alterations in the cancers analysed, we identified mutations in the known pancreatic cancer driver genes: KRAS (88%), TP53 (77%), SMAD4 (29%), CDKN2A (18%) and TGFBR2 (7%; Supplementary Table 2 and Supplementary Data 3 ) [5] , [6] . Homozygous deletions were difficult to assess given the low purity of the samples, but such alterations were identified in CDKN2A in an additional 5% of cases ( Supplementary Data 4 ). We also identified recurrent somatic alterations in genes involved in chromatin regulation or modification, primarily involving the AT-rich interactive domain-containing ARID1A gene (9% of cases) and the histone methyltransferase MLL3 gene (7%; Supplementary Fig. 1 , Supplementary Table 2 and Supplementary Data 3 ) [9] . Six of the alterations in ARID1A were either nonsense or frameshift alterations that were predicted to truncate the protein ( Supplementary Data 3 , Supplementary Fig. 1 ). Mutations in the MLL3 gene included a combination of non-synonymous, nonsense, frameshift and splice-site mutations that occurred in amino acids predicted to be evolutionarily conserved ( Supplementary Data 3 , Supplementary Fig. 1 ). We found somatic frameshift and non-synonymous sequence alterations in the related methyltransferases MLL or MLL2 in eight additional cases. All single-base substitution alterations in these genes were independently validated using the MuTect algorithm [10] . Interestingly, no tumour had more than one gene mutated among the MLL genes suggesting that mutation in any one may be sufficient to confer a selective advantage in neoplastic cells. To determine the expression differences in tumours with alterations in MLL genes, we examined global expression patterns in an independent set of pancreatic tumours with high tumour cellularity where SAGE and sequence data were available [6] (Methods). These analyses indicated that tumours with MLL alterations had expression dysregulation of chromatin-regulating genes, including members of the SWI/SNF chromatin remodelling complex that have been altered in a variety of human cancers, in addition to genes involved in cell cycle progression and other aspects of cellular proliferation ( Supplementary Fig. 2 ). Given the global cellular changes that we and others have found to be regulated by chromatin regulators [11] , [12] , we examined the survival characteristics of patients with mutations in either the MLL or ARID1A genes and found that patients with MLL alterations had a prolonged survival compared with those that were wild type at these loci. Over three quarters (79%) of patients with mutations in MLL , MLL2 or MLL3 were still alive at the time of the analysis (median follow-up of 32 months), while the median survival in patients with wild-type sequences of these genes was 15.3 months ( P =0.0063; log-rank test, Fig. 2 and Supplementary Fig. 3 ). 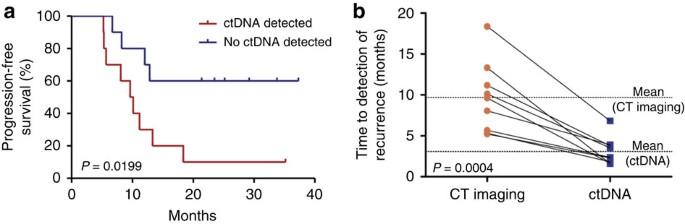Figure 3: Detection of residual disease using computed tomography (CT) imaging and ctDNA analyses. (a) Patients with detectable ctDNA after surgical resection (n=10) were more likely to relapse and die from disease compared with those with undetectable ctDNA (n=10). The median time to recurrence as determined by CT imaging was 9.9 months for individuals with detectable ctDNA and was not reached for those without detectable ctDNA (P=0.0199, log-rank). (b) Comparison between the time to detection of recurrence using ctDNA and standard-of-care CT imaging revealed that the average time to recurrence was 3.1 months for individuals with detectable ctDNA and 9.6 months for those patients with positive imaging results (n=9,P=0.0004, pairedt-test). MLL mutation status was independent of the clinical characteristics measured ( Supplementary Table 3 , P >0.05 for all comparisons by χ 2 - and unpaired t -test) and was found to be an independent prognostic factor ( Supplementary Table 4 , P =0.012, Cox multivariate regression analysis). Patients with alterations in ARID1A had improved survival ( P <0.05, log-rank test) but this observation was limited by a shorter follow-up time in affected individuals. Patients with mutations in any of the chromatin-regulating genes identified had prolonged overall and progression-free survival and these observations were independent of other clinical variables ( P <0.01 for all analyses, Fig. 2 , Supplementary Fig. 3 and Supplementary Table 4 ). Mutation of other epigenetic regulators has been described in cancer and these have been associated with clinical outcome. For instance, improved outcome was reported in patients with DAXX / ATRX alterations in pancreatic neuroendocrine tumours [13] , and a decreased survival in patients with ARID1A and ARID1B mutations in neuroblastoma [14] . Figure 2: Recurrent genetic alterations in pancreatic cancer and their effect on disease outcome. ( a ) Representation of the mutations identified in chromatin modifying and other recurrently mutated genes. Each patient sample is indicated as a grey box with mutations indicated in green or black. ( b ) Analyses of overall survival revealed that patients wild type for MLL gene alterations ( n =87) had a significantly lower median survival compared with those with mutated MLL genes ( n =14; median survival 15.3 months versus not reached respectively, P =0.0063, log-rank test). ( c ) Similar analyses revealed significantly improved survival in patients with mutations in either MLL or ARID1A genes ( n =20) compared with those that were wild type for any of these genes ( n =81). Full size image Non-invasive detection of early-stage pancreatic cancer In parallel to the sequencing analyses of neoplastic tissues, we evaluated the utility of using somatic mutations in ctDNA to identify patients likely to recur after surgical intervention. Through sequencing analyses of tumour samples, we identified somatic mutations that could be used to detect ctDNA in 51 patients from whom plasma was available, largely focusing on alterations in the KRAS gene (Methods). Using digital PCR (dPCR) approaches, we were able to demonstrate that these alterations were detectable in the plasma of 22 patients (43%) at the time of diagnosis, with a specificity of >99.9% (Methods, Supplementary Table 5 ). Consistent with recent reports [15] , [16] , these results suggest that a significant fraction of early-stage pancreatic cancers could be diagnosed non-invasively using approaches that focus on a few specific genetic alterations. dPCR analyses were performed using plasma samples obtained at various time points after surgical resection. These analyses revealed that patients with detectable ctDNA in their plasma were more likely to relapse than those with undetectable alterations ( P =0.02, log-rank test, Fig. 3a ). Disease progression using ctDNA was detected at an average of 3.1 months after surgery compared with 9.6 months using standard computed tomography imaging ( P =0.0004, paired t -test, Fig. 3b ). The presence of ctDNA at the time of diagnosis also provided a predictor of disease recurrence ( P =0.015, log-rank test, Supplementary Fig. 4 ). These analyses suggest that tests to detect sequence alterations in cell-free DNA may provide a highly specific approach for early detection of residual or recurrent disease after surgical resection. Figure 3: Detection of residual disease using computed tomography (CT) imaging and ctDNA analyses. ( a ) Patients with detectable ctDNA after surgical resection ( n =10) were more likely to relapse and die from disease compared with those with undetectable ctDNA ( n =10). The median time to recurrence as determined by CT imaging was 9.9 months for individuals with detectable ctDNA and was not reached for those without detectable ctDNA ( P =0.0199, log-rank). ( b ) Comparison between the time to detection of recurrence using ctDNA and standard-of-care CT imaging revealed that the average time to recurrence was 3.1 months for individuals with detectable ctDNA and 9.6 months for those patients with positive imaging results ( n =9, P =0.0004, paired t -test). Full size image Clinical actionability in pancreatic cancer Given the poor outcome and limited therapeutic options for patients with pancreatic cancer, we investigated whether mutations observed in individual cases may be clinically actionable using existing or investigational therapies. We examined genetic alterations that were associated with (1) FDA-approved therapies for oncologic indications, (2) therapies in published prospective clinical studies and (3) ongoing clinical trials for patients with pancreatic cancer or other tumour types. We also evaluated alterations in five genes in the patients’ germline that may affect cancer predisposition as detection of such changes has important implications for early detection and intervention [17] . Through these analyses, we were able to identify somatic alterations with potentially actionable consequences in over a third (38%) of patients (or up to 98 of the 101 patients (97%) if one includes clinical trials related to alterations in KRAS and TP53 ; Table 1 , Supplementary Table 6 ). These alterations included amplification of the HER-2/neu tyrosine kinase ERBB2 , the serine and threonine kinases AKT1 and AKT2 genes, the cyclin-dependent kinase CDK4 gene and the E3 ubiquitin ligase MDM2 gene ( Supplementary Data 4 ). We also observed non-synonymous somatic mutations in the catalytic domains of the phosphatidylinositol-4,5-bisphosphate 3-kinase, PIK3CA , and the v-kit Hardy-Zuckerman 4 feline sarcoma viral oncogene homologue, KIT ( Supplementary Data 3 ). These alterations were at or nearby previously identified somatic mutations in other human cancers [18] . In addition, we identified three patients with truncating somatic alterations in BRCA2 : two with heterozygous somatic nonsense alterations, a patient with a somatic frameshift alteration and a fourth patient with a germline frameshift in BRCA2 together with a loss of heterozygosity in the matched tumour sample ( Supplementary Data 3 ). Table 1 Clinical actionability of pancreatic cancer*. Full size table These alterations represent potential targets of clinical intervention in pancreatic cancer. Poly(adenosine diphosphate (ADP)-ribose) polymerase inhibitors and DNA-damaging agents such as cisplatin and mitomycin C have been shown to provide a synthetic lethal therapeutic strategy for treatment of cancers with defects in components of the homologous recombination repair pathway, such as BRCA1/2 (refs 19 , 20 , 21 , 22 ). Trastuzumab has demonstrated therapeutic efficacy against GI tumours with ERBB2 amplification [23] and is currently being evaluated in clinical trials for patients with metastatic colorectal cancer [24] . Small-molecule inhibitors have been reported that target proteins or the pathways encoded by the altered genes identified, including PIK3CA , BRAF , AKT1/AKT2 and MDM2 , but these not been evaluated in pancreatic cancer. This study highlights information that may be obtained through the integration of large-scale genomic and clinical analyses in pancreatic cancer. Although careful measures were taken to increase the sensitivity of detecting genetic changes in the tumours and in the circulation of these patients, some alterations may not have been detected due to low tumour purity, limited plasma amounts and low mutant allele frequency. Despite these limitations, these data add to our growing understanding of pancreatic cancer. Through integrated genomic analyses, we have identified MLL genes as markers of improved prognosis, and highlighted clinically actionable alterations in genes not typically evaluated during clinical care of pancreatic cancer patients. Future functional studies will be needed to determine the consequences of MLL gene alterations in tumours and whether mutations in these genes confer equivalent effects. We have also shown that ctDNA in the circulation of pancreatic cancer patients may provide a marker of early detection of subclinical, residual or recurrent disease. These analyses suggest future efforts to evaluate more intensive therapies for patients without MLL alterations or with detectable ctDNA after surgical resection, as well as interventional clinical trials based on actionable alterations observed in pancreatic cancer patients. Samples obtained for sequencing analyses Pancreatic ductal adenocarcinoma tumour specimens and matched germline specimens (from peripheral blood) from 101 patients were used for genomic analyses. Plasma samples were obtained at the time of diagnosis from 44 of these patients as well as seven additional patients ( Supplementary Table 2 ). Informed consent for research use was obtained from all patients at the enrolling institution (University of Pennsylvania, Washington University in St. Louis, Herlev Hospital at the University of Copenhagen) before tissue banking and study approval was obtained. Primary tumour samples for genomic analyses were selected from patients with resectable stage II disease, verified to have ≥10% viable tumour cell content by histopathological assessment and demonstrated to be wild-type for the DAXX / ATRX loci, which have been shown to be associated with improved outcome in patients with pancreatic neuroendocrine tumours [13] . For a subset of cases, plasma samples were obtained at multiple time points after surgery. Flow sorting of aneuploid nuclei Flow sorting of tumour nuclei: individual biopsies were minced with scalpel blades in a petri dish (35 × 100 mm) in NST buffer (146 mM NaCl, 10 mM Tris-HCl, pH 7.5, 1 mM CaCl 2 , 0.5 mM MgSO 4 , 21 mM MgCl 2 , 0.05% bovine serum albumin, 0.2% Nonidet P40 (Sigma)) with 4,6-diamindino-2-phenylindole (4′,6-diamidino-2-phenylindole; 10 μg ml −1 ; Boehringer). The nuclei were then disaggregated with a 25-gauge needle, and subsequently filtered through a 40-μm mesh filter immediately before analyses on an Influx cytometer (Becton-Dickinson, San Jose CA), with ultraviolet excitation and 4′,6-diamidino-2-phenylindole emission collected at >450 nm. We sorted all diploid, aneuploid and tetraploid fractions from each sample. DNA content and cell cycle were analysed using the software programme MultiCycle (Phoenix Flow Systems, San Diego, CA). Sample preparation and next-generation sequencing Sample preparation, library construction, exome and targeted capture, next-generation sequencing and bioinformatics analyses of tumour and normal samples were performed as previously described [8] . In brief, DNA was extracted from frozen or formalin-fixed paraffin-embedded tissue, along with matched blood or saliva samples using the Qiagen DNA formalin-fixed paraffin-embedded tissue kit or Qiagen DNA blood mini kit (Qiagen, CA). Genomic DNA from tumour and normal samples were fragmented and used for Illumina TruSeq library construction (Illumina, San Diego, CA) according to the manufacturer’s instructions or as previously described [14] . In brief, 50 ng–3μg of genomic DNA in 100 μl of TE was fragmented in a Covaris sonicator (Covaris, Woburn, MA) to a size of 150–450 bp. To remove fragments smaller than 150 bp, DNA was purified using Agencourt AMPure XP beads (Beckman Coulter, IN) in a ratio of 1.0 to 0.9 of PCR product to beads twice and washed using 70% ethanol as per the manufacturer’s instructions. Purified, fragmented DNA was mixed with 36 μl of H2O, 10 μl of End-Repair Reaction Buffer, 5 μl of End-Repair Enzyme Mix (cat# E6050, NEB, Ipswich, MA). The 100-μl end-repair mixture was incubated at 20 °C for 30 min, and purified using Agencourt AMPure XP beads (Beckman Coulter, IN) in a ratio of 1.0 to 1.25 of PCR product to beads and washed using 70% ethanol as per the manufacturer’s instructions. To A-tail, 42 μl of end-repaired DNA was mixed with 5 μl of 10 × dA Tailing Reaction Buffer and 3 μl of Klenow (exo-)(cat# E6053, NEB, Ipswich, MA). The 50-μl mixture was incubated at 37 °C for 30 min and purified using Agencourt AMPure XP beads (Beckman Coulter, IN) in a ratio of 1.0 to 1.0 of PCR product to beads and washed using 70% ethanol as per the manufacturer’s instructions. For adaptor ligation, 25 μl of A-tailed DNA was mixed with 6.7 μl of H2O, 3.3 μl of PE-adaptor (Illumina), 10 μl of 5 × Ligation buffer and 5 μl of Quick T4 DNA ligase (cat# E6056, NEB, Ipswich, MA). The ligation mixture was incubated at 20 °C for 15 min and purified using Agencourt AMPure XP beads (Beckman Coulter, IN) in a ratio of 1.0 to 0.95 and 1.0 of PCR product to beads twice and washed using 70% ethanol as per the manufacturer’s instructions. To obtain an amplified library, twelve PCRs of 25 μl each were set up, each including 15.5 μl of H 2 O, 5 μl of 5 × Phusion HF buffer, 0.5 μl of a dNTP mix containing 10 mM of each dNTP, 1.25 μl of dimethylsulphoxide, 0.25 μl of Illumina PE primer #1, 0.25 μl of Illumina PE primer #2, 0.25 μl of Hotstart Phusion polymerase and 2 μl of the DNA. The PCR programme used was: 98 °C for 2 min; 12 cycles of 98 °C for 15 s, 65 °C for 30 s, 72 °C for 30 s; and 72 °C for 5 min. DNA was purified using Agencourt AMPure XP beads (Beckman Coulter, IN) in a ratio of 1.0 to 1.0 of PCR product to beads and washed using 70% ethanol as per the manufacturer’s instructions. Exonic or targeted regions were captured in solution using the Agilent SureSelect v.4 kit or a custom targeted panel for the 111 genes of interest according to the manufacturer’s instructions (Agilent, Santa Clara, CA). The captured library was then purified with a Qiagen MinElute column purification kit and eluted in 17 μl of 70 °C EB to obtain 15 μl of captured DNA library. The captured DNA library was amplified in the following way: Eight 30 μl PCR reactions each containing 19 μl of H 2 O, 6 μl of 5 × Phusion HF buffer, 0.6 μl of 10 mM dNTP, 1.5 μl of dimethylsulphoxide, 0.30 μl of Illumina PE primer #1, 0.30 μl of Illumina PE primer #2, 0.30 μl of Hotstart Phusion polymerase and 2 μl of captured exome library were set up. The PCR programme used was: 98 °C for 30 s; 14 cycles (exome) or 16 cycles (targeted) of 98 °C for 10 s, 65 °C for 30 s, 72 °C for 30 s; and 72 °C for 5 min. To purify PCR products, a NucleoSpin Extract II purification kit (Macherey-Nagel, PA) was used following the manufacturer’s instructions. Paired-end sequencing, resulting in 100 bases from each end of the fragments for exome libraries and 150 bases from each end of the fragment for targeted libraries, was performed using Illumina HiSeq 2000/2500 and Illumina MiSeq instrumentation (Illumina, San Diego, CA). Analysis of next-generation sequencing data Somatic mutations were identified using VariantDx [8] custom software for identifying mutations in matched tumour and normal samples. Before mutation calling, primary processing of sequence data for both tumour and normal samples were performed using Illumina CASAVA software (v1.8), including masking of adapter sequences. Sequence reads were aligned against the human reference genome (version hg18) using ELAND with additional realignment of select regions using the Needleman–Wunsch method [25] . Candidate somatic mutations, consisting of point mutations, insertions and deletions were then identified using VariantDx across the either the whole exome or regions of interest. VariantDx examines sequence alignments of tumour samples against a matched normal while applying filters to exclude alignment and sequencing artifacts. In brief, an alignment filter was applied to exclude quality failed reads, unpaired reads and poorly mapped reads in the tumour. A base quality filter was applied to limit inclusion of bases with reported phred quality score >30 for the tumour and >20 for the normal. A mutation in the tumour was identified as a candidate somatic mutation only when (i) distinct paired reads contained the mutation in the tumour; (ii) the number of distinct paired reads containing a particular mutation in the tumour was at least 2% of the total distinct read pairs for targeted analyses and 10% of read pairs for exome and (iii) the mismatched base was not present in >1% of the reads in the matched normal sample as well as not present in a custom database of common germline variants derived from dbSNP and (iv) the position was covered in both the tumour and normal. Mutations arising from misplaced genome alignments, including paralogous sequences, were identified and excluded by searching the reference genome. Candidate somatic mutations were further filtered based on gene annotation to identify those occurring in protein coding regions. Functional consequences were predicted using snpEff and a custom database of CCDS, RefSeq and Ensembl annotations using the latest transcript versions available on hg18 from UCSC ( https://genome.ucsc.edu/ ). Predictions were ordered to prefer transcripts with canonical start and stop codons and CCDS or Refseq transcripts over Ensembl when available. Finally, mutations were filtered to exclude intronic and silent changes, while retaining mutations resulting in missense mutations, nonsense mutations, frameshifts or splice-site alterations. A manual visual inspection step was used to further remove artifactual changes. In addition, all sequence data from tumours that harboured single-base substitutions in MLL , MLL2 , MLL3 and ARID1A genes were independently analysed using MuTect algorithm [10] to confirm the presence of these alterations. Analysis without a matched normal sample For the identification of putative somatic mutations without a matched normal, additional filters were applied. First, mutations present in an unmatched normal sample, sequenced to a similar coverage and on the same platform as the matched normal, were removed. Second, alterations reported in the 1000 Genomes project, present in >1% of the population or listed as Common in dbSNP138 were filtered. Clinical actionability analyses We selected 200 well characterized genes with potential clinical significance and assessed the level of evidence for clinical actionability in three ways. First, we determined which of the genes were associated with FDA-approved therapies ( http://www.fda.gov/Drugs/ ). Second, we carried out a literature search to identify published prospective clinical studies pertaining to genomic alterations of each gene and their association with outcome for cancer patients. Genes that served as targets for specific agents or were predictors of response or resistance to cancer therapies when mutated were considered actionable. Third, we identified clinical trials ( http://clinicaltrials.gov/ ) that specified altered genes within the inclusion criteria and were actively recruiting patients in August 2014. In all cases, the tumour type relevant to the FDA approval or studied in the clinical trials was determined to allow the clinical information to be matched to the mutational data by both gene and cancer type. Statistical analyses of clinical and genetic data Unpaired t -test and χ 2 -test were employed to compare mutation status of MLL genes among different groups with different clinical and pathological characteristics. Curves for overall survival and progression-free survival (calculated as the time from diagnosis to disease progression) were constructed using the Kaplan–Meier method and compared between groups using the log-rank test. Cox proportional hazards regression analysis was used to determine which independent factors jointly had a significant impact on overall survival. All P values were based on two-sided testing and differences were considered significant at P <0.05. Passenger probabilities were calculated using the binomial test adjusted for gene sizes and corrected for multiple comparisons. Genes that were recurrently mutated within the comprehensive exome analysis (≥2 cases) were considered. Statistical analyses of clinical and genetic features were performed with SPSS version 22 for windows, while conservation of specific genomic positions was evaluated using phyloP software [26] . Digital PCR analyses KRAS , BRAF or PIK3CA somatic point mutations were identified through sequencing analysis of tumour tissues. In cases with matched plasma samples, point mutations were detected in the plasma using droplet digital PCR (ddPCR) using the BioRad QX200 Droplet Digital PCR System (Hercules, CA). In brief, specific ddPCR assays for each point mutation were obtained from BioRad (Hercules, CA) and applied to assess the mutant allele fraction (mutant genomic equivalents/total genomic equivalents). Before analysis of each point mutation in the patient plasma sample, a panel of at least 160 normal control analyses was used to confirm the mutation specificity of the assay. In addition, control samples of wild-type DNA were included in each analysis. Gene expression analyses We assessed differential expression between SAGE libraries harbouring an indel, missense or nonsense mutation ( n =5) in MLL-related genes ( MLL , MLL2 , MLL3 and MLL5 ) and those without a mutation ( n =24) as previously described [27] . Our analysis used the R implementation of this model ( http://bioinformatics.mdanderson.org/main/Publications:Baggerly2003a ). Tags having a low marginal variance ( n =4,733) across all 29 standardized libraries were excluded. To assess the extent to which pathways were upregulated or downregulated in the mutated versus non-mutated samples, we assigned genes to a set of 297 curated pathways. Pathways for which three or fewer genes were assigned were filtered from subsequent analyses ( n =255). For each of the 42 remaining pathways, we computed the sum of the t -statistics scaled by the square root of the number of genes belonging to the pathway. In addition, we used a competitive enrichment strategy [28] and implemented in the R package limma version 3.22.5 (ref. 29 ). Specifically, we assessed whether the t -statistic ranks of a given gene set was significantly higher than randomly selected genes not in the set. We repeated this procedure for each of the 42 gene sets that passed the nonspecific filters discussed above. All statistical analyses for SAGE pre-processing and gene set enrichment analyses were performed in R version 3.1.2 ( http://www.R-project.org ). Accession codes: Sequence data have been deposited at the European Genome-phenome Archive (EGA), which is hosted at the European Bioinformatics Institute (EBI), under study accession EGAS00001001257. How to cite this article: Sausen, M. et al . Clinical implications of genomic alterations in the tumour and circulation of pancreatic cancer patients. Nat. Commun. 6:7686 doi: 10.1038/ncomms8686 (2015).